Atomic layer lithography of wafer-scale nanogap arrays for extreme confinement of electromagnetic waves Squeezing light through nanometre-wide gaps in metals can lead to extreme field enhancements, nonlocal electromagnetic effects and light-induced electron tunnelling. This intriguing regime, however, has not been readily accessible to experimentalists because of the lack of reliable technology to fabricate uniform nanogaps with atomic-scale resolution and high throughput. Here we introduce a new patterning technology based on atomic layer deposition and simple adhesive-tape-based planarization. Using this method, we create vertically oriented gaps in opaque metal films along the entire contour of a millimetre-sized pattern, with gap widths as narrow as 9.9 Å, and pack 150,000 such devices on a 4-inch wafer. Electromagnetic waves pass exclusively through the nanogaps, enabling background-free transmission measurements. We observe resonant transmission of near-infrared waves through 1.1-nm-wide gaps ( λ /1,295) and measure an effective refractive index of 17.8. We also observe resonant transmission of millimetre waves through 1.1-nm-wide gaps ( λ /4,000,000) and infer an unprecedented field enhancement factor of 25,000. Subwavelength confinement of optical energy has been demonstrated using metal particles [1] , [2] , [3] , [4] , [5] , [6] , holes [7] , [8] , [9] , slits [9] , [10] , [11] , gaps [12] , [13] , [14] and tips [15] . The greatest degree of confinement is obtained within a nanometre-scale gap between two metal surfaces [2] , [4] , [16] . Point-like nanometric junctions have been created using aggregates of noble-metal nanoparticles [2] , [4] , [16] , electromigration [17] , electron-beam (e-beam) lithography [18] or scanning probes [19] , but these methods cannot be used for fabricating devices with arbitrary geometries and Ångstrom-scale dimensions over a large area. Furthermore, the amount of light that can be coupled from free space into these point-like junctions is limited, due to the size mismatch with the optical wavelength. Transmission measurements on these point-like junctions are impractical, because of the large background of light that passes by next to the junction. These challenges become even greater at longer wavelengths. In particular, squeezing terahertz (THz) waves into one-nanometre-scale gaps would lead to extremely high field enhancements, but exploiting resonances at THz frequencies will require the nanogap to be extended over millimetre length scales. Here, we demonstrate a simple high-throughput fabrication technique that meets all of the aforementioned challenges. Our method, which we call atomic layer lithography, combines atomic layer deposition (ALD) with ‘plug-and-peel’ metal patterning using adhesive tape. ALD is uniquely suited for the fabrication of sub-nanometre-scale structures, as its self-saturating nature enables conformal deposition of dense, uniform films on metal surfaces with atomic-scale resolution [20] , [21] . Previously, ALD was combined with ion milling to pattern 10-nm gaps along the perimeter of hollow micron-sized metal patterns [22] . As these structures were hollow, transmission measurements still suffered from high background levels; in addition, the dimensions of these structures were not suitable for THz studies. We have therefore developed a new planarization scheme to remove any hollow structures other than the nanogaps themselves. We use this technique to produce nanogap structures with thicknesses of less than 1 nm in opaque metal films. Furthermore, the resulting nanogap extends uniformly along a millimetre-scale loop, allowing us to exploit strong THz resonances. Wafer-scale atomic layer lithography of 1-nm-wide gaps Our processing scheme is illustrated in Fig. 1a–d . First, trenches with the desired geometries are patterned in a substrate using standard patterning techniques, such as optical lithography, e-beam lithography or focused-ion-beam (FIB) milling. The patterned substrate is then coated conformally with Al 2 O 3 via ALD at a typical growth rate of 1–2 Å per cycle. The trenches, now overcoated with the Al 2 O 3 film, are subsequently filled with metal by directional evaporation (the ‘plug’ shown in Fig. 1b ). The plug can be of a different material than the initial substrate. It is crucial that the sidewall of the first layer be vertical, so that there is a discontinuity between the first layer and the second. This makes it possible to peel off the metal film atop the substrate using a standard adhesive tape (single-sided Scotch tape), leaving behind planarized metal plugs that are isolated from the substrate by the Al 2 O 3 film. As the adhesive is in contact only with the second metal layer, the process does not leave any residue on the sample. Although standard lithography defines the overall footprint of the structures, the gap size is independently controlled by ALD, giving Ångstrom-scale lateral resolution along the entire contour of structures. Details on the sample fabrication method are given in the Methods section. 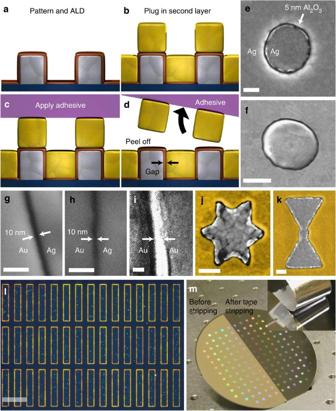Figure 1: Wafer-scale atomic layer lithography. (a) A patterned substrate is conformally coated with a thin layer of insulator (Al2O3) using ALD. (b) A subsequent metal evaporation embeds metal plugs in the substrate. (c,d) Excess metal atop the substrate is removed using an adhesive. (e) Top-view scanning electron micrograph (SEM) of a 5-nm-wide annular gap in a 200–nm–thick Ag film. (f) SEM taken from the bottom side of the structure by stripping it from the substrate. (g) Top-view SEM of a 10-nm-wide Al2O3layer between Ag and Au. (h) Cross-sectional SEM of a 10-nm-wide Al2O3layer between Ag and Au. (i) Cross-sectional TEM of a 9.9-Å-wide Al2O3layer between two Au layers. Colourized top-view SEM of (j) star, and (k) bowtie milled with FIB in a 200 nm-thick Au film on a glass substrate. These patterns were filled with 200-nm-thick Ag plugs with 10-nm-thick Al2O3layers in between. (l) Optical micrograph of a silver nanogap sample (gap size=5 nm; metal thickness=150 nm; total ring length=0.7 mm; total image area=1.6 mm × 1.0 mm). Approximately 150,000 rectangles are patterned over an entire 4-inch glass wafer using standard photolithography. (m) Half of a Si wafer is planarized using adhesive tape (inset), creating a wafer-scale array of Ag plugs in an Si wafer with nanogaps. Scale bars: (e) 300 nm; (f) 300 nm; (g) 50 nm; (h) 50 nm; (i) 1 nm; (j) 300 nm; (k) 300 nm; (l) 0.2 mm. Figure 1: Wafer-scale atomic layer lithography. ( a ) A patterned substrate is conformally coated with a thin layer of insulator (Al 2 O 3 ) using ALD. ( b ) A subsequent metal evaporation embeds metal plugs in the substrate. ( c , d ) Excess metal atop the substrate is removed using an adhesive. ( e ) Top-view scanning electron micrograph (SEM) of a 5-nm-wide annular gap in a 200–nm–thick Ag film. ( f ) SEM taken from the bottom side of the structure by stripping it from the substrate. ( g ) Top-view SEM of a 10-nm-wide Al 2 O 3 layer between Ag and Au. ( h ) Cross-sectional SEM of a 10-nm-wide Al 2 O 3 layer between Ag and Au. ( i ) Cross-sectional TEM of a 9.9-Å-wide Al 2 O 3 layer between two Au layers. Colourized top-view SEM of ( j ) star, and ( k ) bowtie milled with FIB in a 200 nm-thick Au film on a glass substrate. These patterns were filled with 200-nm-thick Ag plugs with 10-nm-thick Al 2 O 3 layers in between. ( l ) Optical micrograph of a silver nanogap sample (gap size=5 nm; metal thickness=150 nm; total ring length=0.7 mm; total image area=1.6 mm × 1.0 mm). Approximately 150,000 rectangles are patterned over an entire 4-inch glass wafer using standard photolithography. ( m ) Half of a Si wafer is planarized using adhesive tape (inset), creating a wafer-scale array of Ag plugs in an Si wafer with nanogaps. Scale bars: ( e ) 300 nm; ( f ) 300 nm; ( g ) 50 nm; ( h ) 50 nm; ( i ) 1 nm; ( j ) 300 nm; ( k ) 300 nm; ( l ) 0.2 mm. Full size image Figure 1e–h depicts scanning electron micrographs of 5-nm-thick annular gaps formed in Ag films and a 10-nm gap formed between Au and Ag. Transmission electron microscopy (TEM) was used to verify the thickness of a 9.9-Å-thick Al 2 O 3 layer on the sidewall of a vertical Au/Al 2 O 3 /Au nanogap ( Fig. 1i ). Figure 1j,k demonstrates that nanogaps with aspect ratios greater than 200 can be formed along the contours of arbitrary patterns. The yield of the plug-and-peel process for a wafer-scale array of metal/Al 2 O 3 /metal nanogap structures ( Fig. 1l,m ) is over 90%. Furthermore, even if the lateral sidewalls display some residual roughness from the initial patterning process, the conformal ALD coating ensures that the nanogaps are uniform in thickness and electrically insulating (see Supplementary Fig. S1 ). A particularly notable feature of our technique is that it can readily form a 1-nm-wide vertical gap along a millimetre-long loop ( Fig. 1l ), as required for resonant transmission of millimetre waves. Because the array of rectangles is patterned by standard photolithography, it was possible to pack approximately 150,000 structures on a 4-inch wafer. Optical characterization of nanogaps To prove that uniform nanogaps are formed through the entire film thickness, we measured optical transmission spectra through a series of nanogaps arranged in rectangular loops with varying lateral dimensions in optically thick Au and Ag films (see Methods for experimental details). As the gaps are oriented vertically, it is straightforward to measure transmission simultaneously through an array of nanogaps simply by imaging the sample under white-light illumination in an optical microscope ( Fig. 2a ). In this configuration, the nanogaps act as metal–insulator–metal (MIM) waveguides, and only the lowest-order, transverse magnetic mode in the waveguide is expected to be excited. This mode is excited only by light polarized perpendicular to the gap [12] , as verified experimentally ( Fig. 2a ). 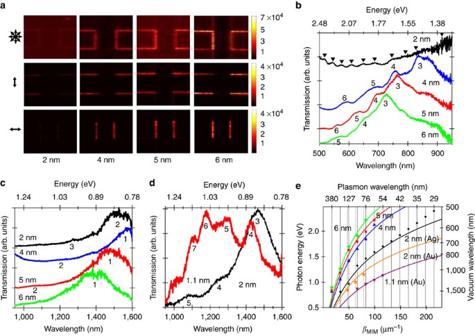Figure 2: Optical transmission measurements through nanogaps. (a) Optical micrograph of white-light transmission through Al2O3-filled nanogaps in 190-nm-thick Ag films. Two adjacent rectangles from the array inFig. 1lare shown. The illumination is unpolarized (row 1), vertically polarized (row 2) and horizontally polarized (row 3). The widths of the gaps are indicated below each column. The colour scale bars on the right show charge-coupled device counts. (b) Measured transmission spectra through nanogaps in Ag at visible wavelengths. (c) Measured transmission spectra through nanogaps in Ag at NIR wavelengths. Spectra from 2, 4, 5 and 6 nm gaps in (b,c) are offset vertically for ease of comparison. (d) Measured transmission spectra at NIR wavelengths through a 1.1-nm gap in a 190-nm-thick Au film and a 2-nm gap in a 200-nm-thick Au film. Numbers in (b–d) are the mode orders of FP resonances in the nanogap waveguides. Triangles in (b) indicate FP resonance positions for 2-nm gaps; from right to left, modes 4–13 are indicated. (e) Dispersion relations of gap-plasmon modes in MIM nanogaps. The solid curves are theoretical dispersion curves for different gap sizes and materials. The markers are measured resonance peaks from MIM nanogap waveguides (b–d). The vertical solid grey grid lines denote the wavenumbers of modes 1–13, from left to right, for a cavity length of 190 nm. The vertical dashed gray grids mark the wavenumbers of modes 3, 4 and 5 for a cavity length of 200 nm. Figure 2: Optical transmission measurements through nanogaps. ( a ) Optical micrograph of white-light transmission through Al 2 O 3 -filled nanogaps in 190-nm-thick Ag films. Two adjacent rectangles from the array in Fig. 1l are shown. The illumination is unpolarized (row 1), vertically polarized (row 2) and horizontally polarized (row 3). The widths of the gaps are indicated below each column. The colour scale bars on the right show charge-coupled device counts. ( b ) Measured transmission spectra through nanogaps in Ag at visible wavelengths. ( c ) Measured transmission spectra through nanogaps in Ag at NIR wavelengths. Spectra from 2, 4, 5 and 6 nm gaps in ( b , c ) are offset vertically for ease of comparison. ( d ) Measured transmission spectra at NIR wavelengths through a 1.1-nm gap in a 190-nm-thick Au film and a 2-nm gap in a 200-nm-thick Au film. Numbers in ( b – d ) are the mode orders of FP resonances in the nanogap waveguides. Triangles in ( b ) indicate FP resonance positions for 2-nm gaps; from right to left, modes 4–13 are indicated. ( e ) Dispersion relations of gap-plasmon modes in MIM nanogaps. The solid curves are theoretical dispersion curves for different gap sizes and materials. The markers are measured resonance peaks from MIM nanogap waveguides ( b – d ). The vertical solid grey grid lines denote the wavenumbers of modes 1–13, from left to right, for a cavity length of 190 nm. The vertical dashed gray grids mark the wavenumbers of modes 3, 4 and 5 for a cavity length of 200 nm. Full size image The spectra of light transmitted through the nanogaps show a series of peaks at visible and near-infrared (NIR) wavelengths ( Fig. 2b–d ), which correspond to Fabry–Pérot (FP) resonances [12] , [23] : light travelling in the MIM waveguide is partially reflected at the upper and lower surfaces of the metal film, forming a resonator whose length, L , is determined by the film thickness. The resonances occur when the following condition is satisfied: where β MIM is the propagation constant in the MIM waveguide, m is the integer FP mode number and Δ φ 1,2 describe phase shifts due to reflection at the two end faces of the cavity. To obtain a simple analytical model, we ignore these phase shifts, which are expected to be small due to the large effective-index mismatch between the waveguide and free space. We can then use equation (1) to map out the dispersion relation of the MIM waveguides, provided that we know which mode number, m , corresponds to a given transmission peak. The mode number was determined by comparing the measured data to finite-difference time-domain (FDTD) simulations (not shown), and resonance peak positions were obtained by fitting Lorentzian peaks to the measured spectra. As shown in Fig. 2e , experimental data from the Au and Ag nanogaps are in good agreement with theoretical dispersion relations; deviations for large wavenumbers may be due to the neglect of the phase shifts upon reflection or due to errors or variations in the measured thickness of the metal film. The dispersion curves indicate that light with a free-space wavelength of 517 nm, when confined to a 2-nm Al 2 O 3 gap in Ag, takes on a plasmon wavelength λ SP =29 nm; this corresponds to an effective refractive index of 17.8, the highest index yet reported in the visible spectral range. THz time-domain spectroscopy and field enhancement Although the film thickness determines FP resonances at optical frequencies, the horizontal dimension of the loop determines in-plane resonances at THz frequencies ( Fig. 3a ). When the nanogaps are irradiated with THz waves, induced current charges the capacitor formed by the sidewalls of the nanogap. For smaller gaps, Coulomb attraction brings opposite charges closer to the sidewalls and generates a field enhancement that is inversely proportional to the gap size [11] , [24] . Previously, a field enhancement of 1,000 was experimentally demonstrated for a non-resonant 70-nm-wide slit [11] , and much larger enhancements are expected for 1-nm-wide gaps. Indeed, two-dimensional (2D) FDTD simulation using the dielectric function for a Drude model of Ag predicts an electric-field enhancement factor of 7,800 at a wavelength of λ= 4 mm ( Fig. 3b ) and 10,000 at λ =5.4 mm for 1-nm gaps (see the Methods for details on the FDTD calculations). 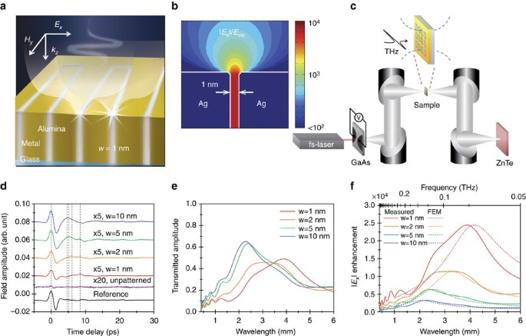Figure 3: Giant THz field enhancements in nanogap ring structures. (a) Illustration of THz waves being funneled through nanogaps arranged in rectangular rings. (b) Calculated electric-field enhancement within a 1 nm-wide slit in an Ag film at the wavelength of 4 mm. Fields were determined using a 2D FDTD simulation, approximating the dielectric function of Ag using the Drude model. Fields can be seen to be concentrated entirely within the gap. (c) Experimental setup for THz-TDS consisting of a femtosecond Ti-sapphire laser, GaAs emitter, nanogap sample and ZnTe electro-optic detector. (d) Time traces for transmitted THz waves through the bare substrate (reference), unpatterned Ag film and nanogap samples with the gap sizes of 1, 2, 5 and 10 nm. The time traces are offset along the vertical axis for clarity. (e) Fourier-transformed electric-field amplitude, normalized by the reference signal, as a function of wavelength. (f) Electric-field enhancement, normalized by the coverage ratio of nanogaps with the gap sizes ofw=1, 2, 5 and 10 nm. Solid lines indicate measured fields, determined by THz-TDS. The ringing at wavelengths below 2 mm is due to FP resonances in the glass substrate. Dashed lines indicate calculated transmission spectra, determined by 2D finite element modelling. To allow resonance wavelengths to be compared, peak values of these calculated spectra are set to the peak values of the experimental spectra. Figure 3: Giant THz field enhancements in nanogap ring structures. ( a ) Illustration of THz waves being funneled through nanogaps arranged in rectangular rings. ( b ) Calculated electric-field enhancement within a 1 nm-wide slit in an Ag film at the wavelength of 4 mm. Fields were determined using a 2D FDTD simulation, approximating the dielectric function of Ag using the Drude model. Fields can be seen to be concentrated entirely within the gap. ( c ) Experimental setup for THz-TDS consisting of a femtosecond Ti-sapphire laser, GaAs emitter, nanogap sample and ZnTe electro-optic detector. ( d ) Time traces for transmitted THz waves through the bare substrate (reference), unpatterned Ag film and nanogap samples with the gap sizes of 1, 2, 5 and 10 nm. The time traces are offset along the vertical axis for clarity. ( e ) Fourier-transformed electric-field amplitude, normalized by the reference signal, as a function of wavelength. ( f ) Electric-field enhancement, normalized by the coverage ratio of nanogaps with the gap sizes of w =1, 2, 5 and 10 nm. Solid lines indicate measured fields, determined by THz-TDS. The ringing at wavelengths below 2 mm is due to FP resonances in the glass substrate. Dashed lines indicate calculated transmission spectra, determined by 2D finite element modelling. To allow resonance wavelengths to be compared, peak values of these calculated spectra are set to the peak values of the experimental spectra. Full size image To experimentally probe the THz response of the nanogap waveguides, we performed THz time-domain spectroscopy (TDS) [25] , [26] over a wavelength range of 0.2–6.0 mm (1.5–0.05 THz) on 150-nm-thick Ag samples with gap sizes w =1, 2, 5 and 10 nm (see Fig. 3c and the Methods section for experimental details). Figure 3d shows that the period of the second oscillation on the transmitted THz time traces increases from 7.7 to 13 ps as the gap size decreases from 10 to 1 nm. These distortions of transmitted THz pulses correspond to resonance peaks in the spectral domain. By taking the Fourier transform of these time-domain traces, we determined that the amplitude transmittance of the input pulse through an array of 1-nm gaps, which occupy only 0.002% of the chip area, was as high as 50% at the resonance wavelength of ~4 mm ( Fig. 3e ). By contrast, the direct THz transmission through an unpatterned metal film was only 0.1%, indicating very strong field enhancement inside the gap. To quantify the enhancement factor, we use diffraction theory [11] , which is based on the assumption that the field is concentrated exclusively within the gap. This approximation is justified because the dielectric constant of the metal is ~10 6 times larger than that of the dielectric gap at THz frequencies, so that the field intensity in the metal is very small. Using this formalism, we infer field enhancement factors as high as 25,000 ( Fig. 3f , solid line). Details on the determination of enhancement factors are given in the Methods section. This value is even higher than the factor of 10,000 predicted by the 2D FDTD simulations, due to in-plane THz resonances along the 0.7-mm-long contour of each rectangular loop [27] . To verify that the observed transmission resonances are indeed due to these loops (see Supplementary Fig. S3 ), we used 2D finite element modelling to determine the eigenmodes of the ring structures ( Fig. 3f , dotted line). To obtain agreement between the measured and calculated resonance frequencies, it was necessary to use a thickness-dependent dielectric constant for the Al 2 O 3 film [28] , [29] (see the Methods section and Supplementary Fig. S4 for details). This thickness-dependent response has been inferred from electrical transport measurements, but has not previously been considered when treating the optical response of nanometre-scale junctions. We have presented a simple patterning method—atomic layer lithography—based on standard photolithography, ALD and adhesive tape, that enables wafer-scale production of 1-nm nanogap arrays containing approximately 150,000 devices. NIR waves pass through gaps with dimensions as much as 1,295 times smaller than the free-space wavelength, and we measure an effective refractive index at visible frequencies as high as 17.8. Our method has the unique ability to produce nanometre-scale gaps over millimetre-scale contours, enabling resonantly enhanced transmission of THz waves through opaque metal films. Funneling of THz radiation through 1-nm gaps leads to unprecedented field enhancement factors of 25,000, corresponding to intensity enhancement factors of 6.25 × 10 8 . Because the measured transmission passes exclusively through the 1-nm gaps, which occupy <0.002% of the chip area, we can separate light transmitted through the nanogaps from the illumination background even for millimetre-sized beam spots. Pushing the gap dimension towards the Ångstrom scale may become feasible; this would enable wafer-scale investigation of quantum-mechanical and nonlocal effects at optical frequencies [1] , [30] , [31] , [32] , optical rectification [14] and inelastic electron tunnelling excitation of plasmons [33] , [34] . Furthermore, by inserting molecules, nanoparticles or optically active materials in vertically oriented nanogaps, one could dramatically enhance light–matter interactions over a wide spectral range, enabling a new generation of THz detectors [35] and leading to novel nonlinear phenomena [36] . Atomic layer deposition An Al 2 O 3 layer was deposited by ALD at 250 °C on Au substrates and at 50 °C on Ag substrates to avoid unwanted oxidation. Trimethylaluminum and water vapour were sequentially pulsed through the chamber with N 2 purging after each injection. Deposition rates were 1.1 Å per cycle on Au and 1.83 Å per cycle on Ag. The thickness of the Al 2 O 3 film was calibrated using ellipsometry on control wafers placed in the same chamber. Adhesive-tape-based planarization After the ALD step and the deposition of the second metal layer, the metal film atop the substrate was removed by gently contacting the top layer with one-sided Scotch tape and peeling it off. The metal can be cleanly removed because of the poor adhesion between noble metals (Au and Ag) and Al 2 O 3 , and only the top metal film is removed, due to the height difference between the metal inside and outside the patterned area. The peeling process has been successfully performed for patterns that are as large as 1 mm × 5 mm, and leaves behind no residue. TEM sample preparation A lamina of the Au/Al 2 O 3 /Au structure was cut at one side of the rectangular pattern by FIB milling, was picked up using an Omniprobe and was attached to a TEM grid. The lamina was further thinned by FIB milling to <100 nm for imaging by TEM (JEM-ARM200F, JEOL). Optical transmission measurements For transmission measurements at NIR wavelengths, nanogaps were illuminated with an unfiltered halogen lamp through a condenser on an Olympus IX71 inverted microscope and the transmitted light was collected with an Olympus LMPlan IR × 100 objective and imaged on the entrance slit of an Acton SP2300 grating spectrometer equipped with a liquid-N 2 -cooled OMA V InGaAs focal-plane photodiode array (Princeton Instruments). For transmission measurements at visible wavelengths, a Nikon Eclipse inverted microscope, a Newport MS257 imaging spectrometer, and a Princeton Pixis 400 CCD camera were used. Spectra were normalized to the illumination source and a background spectrum was subtracted from all measured spectra. Each spectrum was measured through a single gap and averaged over the length of the gap. Repeatable spectra were obtained from different gaps on the same samples. Nanogap samples for optical transmission measurements were made using standard photolithography (except the spectrum for 2 nm gap in gold film in Fig. 2d , which was taken from a sample made using FIB). Terahertz time-domain spectroscopy We measure the transmission spectra of nanogap rectangular ring arrays in the wavelength range from 0.2 mm (1.5 THz) to 6 mm (0.05 THz) using electro-optic sampling THz-TDS [11] . We use a femtosecond Ti:sapphire laser to illuminate a GaAs emitter with a pulse train of wavelength 780 nm, 80 MHz repetition rate, and 130-fs pulse width. The p -polarized millimetre-wavelength pulses are normally incident on the nanogap ring structure ( Fig. 3c ). The THz waves transmitted through the nanogap are collected using parabolic mirrors (NA=0.32) and detected via electro-optic sampling using a (110)-oriented ZnTe crystal. The nanogap samples used for THz measurements (optical micrographs in Fig. 1l ) were made using standard photolithography, with 1, 2, 5 and 10 nm gaps along 50 × 300 μm 2 rectangular patterns. Finite-difference time-domain simulation for the 1-nm gap sample Figure 3b of the main text shows the results of 2D FDTD calculations for a 1-nm-wide infinite slit, filled with Al 2 O 3 , in an Ag film. To cover the widely different length scales involved, from the millimetre-scale free-space wavelength, λ , to the nanometre-scale gap size, asymptotically varying grid sizes were employed [37] . A 0.25-nm grid size was used near the nanogap, and the grid size gradually becomes larger further away from the nanogap, up to λ /20. A total area of 7.5 × 4.0 mm 2 was simulated. Convergence was confirmed by varying the grid density along each axis by a factor of two, and verifying that calculated field amplitudes changed by <2% over the entire simulation space. The dielectric function of Ag was approximated by the Drude model, , where ε ∞ =1, ω p =1.37 × 10 4 (THz) and γ =27.4 (THz) [38] . We also use a thickness-dependent dielectric constant for the Al 2 O 3 layer, as explained below. Determination of field enhancements To estimate field enhancements from our far-field THz-TDS measurements, we first measured the transmitted electric field at the ZnTe detector through a bare glass substrate with a 3.5 × 3.5 mm 2 reference aperture. We then measured the electric field for the nanogap sample, denoted . The normalized amplitude, t , is defined as the ratio of these two measured amplitudes: . The enhancement of the local electric field within the nanogaps can simply be inferred from t based on the approximation that the metal acts as a perfect electrical conductor (PEC). Although the PEC approximation cannot be used at optical and NIR frequencies, it provides a very good approximation of field enhancements at THz frequencies [11] . The complex refractive index of the metal in the THz regime is very large, on the order of 1,000+1,000 i , which means that penetration of the electric field into the metal is minimal. More quantitatively, for the normally oriented electric fields within the nanogap, the boundary condition D 1x = D 2x means that the field in the metal is weaker than the field in the dielectric by a factor | ε dielectric / ε metal | (see Supplementary Fig. S2 ). At a frequency of 0.1 THz, this factor is ~10 −6 . For our measurements, this is the factor that is important in determining the validity of the PEC approximation, rather than the skin depth. Even if we assume that the field within the metal is uniform, and considering that the area filled with metal is 50,000 times larger than the area of the nanogaps, the error in the field-enhancement calculation obtained using the PEC approximation would be only 50,000/10 6 =5%. The PEC approximation makes it possible to estimate the field enhancement factor using the Kirchhoff integral formalism. Including the effect of the collection optics (NA=0.32) in our THz setup changes the field enhancement only by a few percent, compared with the simple Kirchhoff estimate. We obtain where A aperture is the aperture area and R is the distance from the aperture to the detector. Likewise, where A gap is the total area of the nanogaps and is the unknown, averaged field at the gap. Dividing the two equations, we obtain the field enhancement factor , where . Finite element method simulations of THz resonances in nanogap ring structures We modelled the transmission resonances observed in our THz-TDS measurements ( Fig. 3f in the main text) using finite element method simulations, employing the Wave Eigenmode Analysis tool in COMSOL’s Electromagnetics Module. Non-reflecting boundaries are implemented on the top and bottom edges of the 2D computational window, which includes the cross-section of the Ag/Al 2 O 3 /Ag waveguide on a glass substrate. A grid size of 0.2 nm is used to calculate the field inside the metal and at the nanogap, and the grid size gradually increases away from the gap, reaching a maximum value of λ /20. The entire simulation space is set to λ × λ . The dielectric function of Ag was approximated using the same Drude model as for the FDTD calculations. For a given input frequency, the COMSOL solver calculates the effective refractive index of the MIM waveguide system, n eff , by dividing the free-space wavelength λ 0 by the gap-plasmon wavelength, λ MIM , obtained from the eigenmode solutions. The effective refractive index satisfies where m is the mode number and l is the total length of the MIM ring resonator in the film plane. We consider only the first resonant mode ( m =1). The wavelength-dependent field enhancement is obtained by sweeping the input frequency. Agreement between calculated and measured resonance frequencies was obtained only by using thickness-dependent dielectric constants for the Al 2 O 3 layer. These thickness-dependent dielectric constants have been previously reported [28] , [29] and are believed to result from metal–dielectric interfacial effects, including a combination of field penetration into the metal, strain in the lattice-mismatched Al 2 O 3 layer and surface roughness. Supplementary Fig. S4a shows the effective refractive index of Al 2 O 3 that is used in the calculations. Supplementary Fig. S4b compares the calculated n eff as a function of the gap size using the bulk dielectric constant of 10.5 and those obtained using thickness-dependent dielectric constants; the thickness-dependent values clearly lead to much better agreement with experiment. How to cite this article: Chen, X. et al . Atomic layer lithography of wafer-scale nanogap arrays for extreme confinement of electromagnetic waves. Nat. Commun. 4:2361 doi: 10.1038/ncomms3361 (2013).